Vibrio choleraeuse pili and flagella synergistically to effect motility switching and conditional surface attachment We show that Vibrio cholerae , the causative agent of cholera, use their flagella and mannose-sensitive hemagglutinin (MSHA) type IV pili synergistically to switch between two complementary motility states that together facilitate surface selection and attachment. Flagellar rotation counter-rotates the cell body, causing MSHA pili to have periodic mechanical contact with the surface for surface-skimming cells. Using tracking algorithms at 5 ms resolution we observe two motility behaviours: ‘roaming', characterized by meandering trajectories, and ‘orbiting’, characterized by repetitive high-curvature orbits. We develop a hydrodynamic model showing that these phenotypes result from a nonlinear relationship between trajectory shape and frictional forces between pili and the surface: strong pili–surface interactions generate orbiting motion, increasing the local bacterial loiter time. Time-lapse imaging reveals how only orbiting mode cells can attach irreversibly and form microcolonies. These observations suggest that MSHA pili are crucial for surface selection, irreversible attachment, and ultimately microcolony formation. V ibrio cholerae is a vibroid-shaped gram-negative bacterium found in coastal and brackish waters, and is the causative agent of the diarrhoeal disease cholera [1] , [2] , [3] . Seasonal cholera epidemics occur as environmental conditions become favourable for growth of the native reservoirs of V. cholerae [2] , [4] , [5] . V. cholerae can attach to the surfaces of phytoplankton, zooplankton and crustaceans [4] , [6] as surface-attached biofilm communities [3] , [4] , [6] , [7] , [8] , which are composed of cells adhered to a surface through extracellular polymeric substances that consist primarily of polysaccharides and adhesive proteins [9] , [10] . This biofilm lifestyle affords greater protection from environmental variability, predation and antimicrobials [9] , [11] , [12] . The model organism Pseudomonas aeruginosa reversibly attach to surfaces in a vertical orientation [9] and move along random trajectories with type IV pili (TFP)-driven ‘walking motility’ in the early stages of biofilm formation [13] . These cells can progress to an irreversibly attached state where the cell axis is oriented parallel to the surface. Such horizontal cells can move by TFP-driven ‘crawling’ or ‘twitching’ motility, which has much more directional persistence. Recent work has shown that P. aeruginosa PAO1 cells interact with a network of Psl polysaccharides secreted onto the surface that allows them to self-organise in a manner reminiscent of ‘rich-get-richer’ economies, ultimately resulting in the formation of microcolonies [14] . V. cholerae also use TFP to engage non-nutritive, abiotic surfaces. Despite having three different types of TFP, mannose-sensitive hemagglutinin (MSHA) pili, virulence-associated toxin co-regulated pili and chitin-regulated pili (ChiRP), V. cholerae do not appear to have a twitching surface motility mode [9] , [15] and it is unclear how they form microcolonies. Although V. cholerae lack a twitching mode, it is known that MSHA pili and flagella play important roles in biofilm development; MSHA pili (Δ mshA ) and flagellar (Δ flaA ) mutants require much more time than wild type (WT) to develop into biofilms in static environments [16] . The details, however, are at present also unknown. Here we show that V. cholerae use their polar flagellum and MSHA pili synergistically to scan a surface mechanically before irreversible attachment and microcolony formation. Flagellum rotation causes the Vibrio cell body to counter-rotate along its major axis, which in principle allows MSHA appendages to have periodic mechanical contact with the surface for surface-skimming cells. We apply cell-tracking algorithms to high-speed movies of V. cholerae taken at 5 ms resolution to reconstruct the motility history of every cell that comes within 1 μm of the surface in a 160 μm × 120 μm field of view, and observe two distinct near-surface motility modes: ‘roaming’ motility, which is characterized by long persistence length trajectories, and ‘orbiting’ motility, which is characterized by near-circular trajectories with well-defined radii. In both motility modes cells move in an oblique direction that deviates strongly from the major cell axis and have strong nutations along the trajectory. These motility behaviours are ablated in Δ mshA and Δ flaA mutants. We develop a hydrodynamic model to show that the bifurcation into these two surface motility phenotypes is a consequence of the highly nonlinear dependence of trajectory shape on frictional forces between MSHA pili and the surface: cells naturally loiter over regions that interact more strongly with MSHA pili, due to orbiting motility. This simple theoretical description agrees remarkably well with the observed trajectories, including the distribution of velocities, and the direction of motion relative to the major axis of the cells. Interestingly, V. cholerae cells that eventually attach exhibit a distribution of intermittent pauses during the preceding orbiting motility. Both the frequency and duration of these pauses are strongly suppressed when cells are incubated with a non-metabolisable mannose derivative to saturate MSHA pili binding. Moreover, the sites of irreversible attachment correlate with the positions of eventual microcolonies, which indicates that purely TFP-driven motility plays a minor role in determining positions of microcolonies, unlike the case for P. aeruginosa . These observations suggest that MSHA pili–surface binding is crucial to arresting cell motion during near-surface swimming and the transition to irreversible attachment and microcolony formation. Near-surface motility of WT cells Cells must first swim to a surface before they can attach and the hydrodynamics of these interactions have been studied extensively [17] , [18] , [19] , [20] , [21] , [22] , [23] . Bacteria swimming near surfaces experience hydrodynamic forces that both attract them towards the surface and cause them to swim in circular trajectories [15] , [18] , [20] , [24] , [25] . Both polytrichous Escherichia coli and monotrichous vibrios have been observed to swim in clockwise (CW) circular patterns near surfaces [15] , [18] , [20] , [24] , [26] . Hydrodynamic models show that a torque on the cell body is induced by viscous drag forces felt by the flagellum as it sweeps past a surface; this surface-induced torque deflects the swimming direction of cells into curved CW paths [20] . V. cholerae are among the fastest bacterial swimmers. They are equipped with a Na + motor that enables them to swim at speeds up to 100 μm s −1 (ref. 27 ). We record bright-field movies using a high-speed camera and use cell-tracking algorithms [28] (Methods) to track and analyze the motion of V. cholerae on glass at different times after inoculation. The trajectories of the centroids of all WT cells tracked in this period are shown in Fig. 1a . Tracking all cells in the field of view reveals many cells that appear to travel in tight orbital paths. A large number of mobile bacteria visit the surface, but relatively few attach irreversibly during this initial period. A binary image of the stationary cells taken during the same period and location is shown Fig. 1b . 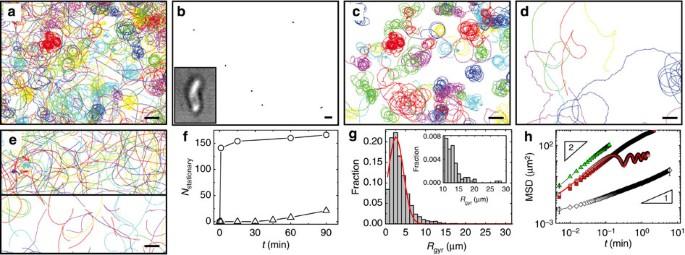Figure 1: Near-surface trajectories generated by cell tracking and analysis. (a) WT trajectories extracted from a high-speed movie of 100 s at 5 ms resolution during the first 5 min after inoculation. Different tracks are represented by different colours. Scale bars, 10 μm and applies toa–e. (b) Binary image of stationary, surface-adherent cells at the end of the 100 s movie. (inset) Bright-field image of aV. choleraecell. Width of the image, 2 μm. (c) Subset of the population inafiltered for cells exhibiting orbiting motility. (d) Subset of the population inafiltered for cells exhibiting roaming motility. (e) ΔmshAmutant trajectories extracted from a high-speed movie of 100 s at 5 ms resolution during the first 5 min after inoculation. (e, lower) Lower half of the same field of view showing only a subset of all cells to enable better visualization. (f) Number of surface-adhered cells as a function of time for WT (○) and ΔmshA(Δ) with same initial cell number density. (g) Histogram ofRgyrfor all WT tracks ina(N=3315). The (red) line is a fit to a normal distribution centred at 2.6 μm. (inset) Expanded view of the fraction ofRgyr>10 μm. (h) MSD versus time for representative WT orbiting (○) and roaming cells (□). The red line is a model fit to the MSD of the orbiting cell. Average MSD of all ΔmshAmutants (Δ;NΔmshA=2,030) and ΔflaAmutants (◊;NΔflaA=6). Error bars represent 1 s.d. The numbers represent the slopes of the two lines. Figure 1: Near-surface trajectories generated by cell tracking and analysis. ( a ) WT trajectories extracted from a high-speed movie of 100 s at 5 ms resolution during the first 5 min after inoculation. Different tracks are represented by different colours. Scale bars, 10 μm and applies to a – e . ( b ) Binary image of stationary, surface-adherent cells at the end of the 100 s movie. (inset) Bright-field image of a V. cholerae cell. Width of the image, 2 μm. ( c ) Subset of the population in a filtered for cells exhibiting orbiting motility. ( d ) Subset of the population in a filtered for cells exhibiting roaming motility. ( e ) Δ mshA mutant trajectories extracted from a high-speed movie of 100 s at 5 ms resolution during the first 5 min after inoculation. ( e , lower) Lower half of the same field of view showing only a subset of all cells to enable better visualization. ( f ) Number of surface-adhered cells as a function of time for WT ( ○ ) and Δ mshA (Δ) with same initial cell number density. ( g ) Histogram of R gyr for all WT tracks in a ( N =3315). The (red) line is a fit to a normal distribution centred at 2.6 μm. (inset) Expanded view of the fraction of R gyr >10 μm. ( h ) MSD versus time for representative WT orbiting ( ○ ) and roaming cells (□). The red line is a model fit to the MSD of the orbiting cell. Average MSD of all Δ mshA mutants (Δ; N Δ mshA =2,030) and Δ flaA mutants ( ◊ ; N Δ flaA =6). Error bars represent 1 s.d. The numbers represent the slopes of the two lines. Full size image To extract the orbital motion evident in the WT ensemble (see Fig. 1a ), we limit our search to mobile cells, defined as cells that travel a minimum distance of at least one cell length, that are visible for at least 1 s, and have a mean-squared displacement (MSD) slope>1 (Methods). The MSD as a function of time interval, t , is a statistical measure of the average shape of the trajectories. The MSD( t ) of purely diffusive particles generally has a slope of 1, while that of purely ballistic motion has a slope of 2. We filter this database of mobile-cell trajectories using a threshold value of the radius of gyration ( R gyr ), which is a statistical measure of the spatial extent of an ensemble of points [29] . The R gyr is defined as , where N is the number of points in the track, is the position vector of the i th point on the trajectory, and is the centre-of-mass of all points. For a perfect circle of radius, r , the R gyr = r . R gyr gives accurate information about the overall extent of the trajectory at the longest observation time, whereas the MSD gives information about displacements between points at fixed time intervals and is more suitable for short time lags. Qualitatively, two types of trajectories are observed: one with tight near-circular orbits with high curvatures (‘orbiting’, Fig. 1c ) and one with long directional persistence and small curvatures (‘roaming’, Fig. 1d ). In both cases, the direction of motion seems to be exclusively in the CW sense. From three separate trials, we observe that all cells orbit in the CW direction ( N =255, 149 and 352). We search for S-shaped trajectories among the roaming cells, which is a signature of CW to CCW rotation, and exclude segments of trajectories where cells have clearly made surface attachment. In three trials, we find no such trajectories ( N =17, 8 and 7). The distribution of R gyr extracted for all WT trajectories shows a distinct peak at ~3 μm with a long tail of larger values (see Fig. 1g ). We fit the data to a normal distribution centred at 2.6 μm with a s.d. of 1.9, and set a threshold value of R gyr =8 μm at the upper end of the orbital motility behaviour. Based on R gyr , we classify cells as either ‘orbiting’ ( R gyr <8 μm) or ‘roaming’ ( R gyr >8 μm). Orbiting cells undergo periodic orbital motion with tight distributions of radii and have orbital centres that slowly diffuse on the surface, so that these cells tend to loiter over the same area. In contrast to the behaviour of cells executing ‘orbiting’ motility, cells undergoing ‘roaming’ motility travel over large areas of the surface along trajectories with extremely polydisperse curvatures. It should be noted that the radii of trajectories of near-surface swimming E. coli are significantly larger, with r ≈20–30 μm, and have more variability compared with those observed in Vibrio ‘orbiting’ motility [20] , [24] , [30] . Near-surface motility of mshA and flaA mutants To see that orbiting and roaming motility are qualitatively different, we calculate the MSD ( t ) and compare representative WT cells exhibiting roaming and orbiting behaviour, respectively, with that of Δ mshA and Δ flaA mutants. For t ranging from 5 to 100 ms both WT subpopulations have slopes of ~2. At longer t , the slope of the MSD for roaming cells gradually tends towards 1, consistent with the random meandering nature of the movement at sufficiently long timescales. In contrast, the MSD of the orbiting subpopulation shows a strong oscillation that corresponds to their orbit period. The upward trend at t >100 ms of this oscillation reflects the fact that centre of the orbit itself is weakly diffusive ( Fig. 1h , □ and ○ ). Similar oscillations in the MSD ( t ) have been observed in systems of self-propelled colloids that have a strong rotational component to their motion [31] . We fit the MSD for this orbiting cell and extract a rotational diffusion constant (red line, Fig. 1h ; Supplementary Note , Supplementary Fig. 1 and Supplementary Table 1 ). Since the Δ flaA mutants lack flagella, they simply diffuse across the surface until their MSHA pili attach. As expected, the slope of the MSD for unattached Δ flaA mutants is ~1 ( Fig. 1h , ◊ ). In contrast, the swimming trajectories of Δ mshA mutants are unhindered by attachment to the surface and represent the opposite extreme; their slopes are nearly 2 for all t ( Fig. 1h , Δ), generally indicating ballistic motion. The MSDs demonstrate that at any t , on average, the Δ mshA mutants travel farther and spend less time hovering near the surface than WT. The roaming and orbiting WT subpopulations are found between the two extremes of Δ flaA and Δ mshA . Angle of motion Interactions between MSHA pili and surfaces significantly influence trajectories and time spent over a given patch of surface; consistent with this, tracks of Δ mshA mutants are straighter than WT (see Fig. 1e ). To achieve high-curvature trajectories along a surface, cells must exhibit significant off-axis components to their motion and non-zero angles between the body axis and the direction of motion (see inset in Fig. 2 for schematic). Although current hydrodynamic models for near-surface swimming bacteria can generate circular trajectories, they typically consider only the angle between the surface and the cell’s body axis [18] , [20] , [21] and not the angle between the body axis and direction of motion. In our experiments, the depth of focus is shallow (≤0.2 μm); therefore, for cells that are in focus, the angle between the surface and the body axis is small. We measure the instantaneous orientation and direction of motion of all cells. We monitor the angle between the body axis and the direction of motion, θ , at each point along the trajectories and average it over the entire track (‹ θ ›). We find that the histogram of ‹ θ › for Δ mshA mutants has a single peak centred at ~15°, implying that they are swimming nearly along their body axis. The histogram of ‹ θ › for WT has a similar peak centred at ~15° but in addition, it has a second peak centred at ~45° (see Fig. 2 ). The first peak indicates that there is a subset of the WT cells that behave similar to Δ mshA mutants, and do not interact strongly with the surface. In contrast, the WT subpopulation with large angular deflections centred at ~45° includes both the orbiting and roaming populations (see Fig. 2 ). 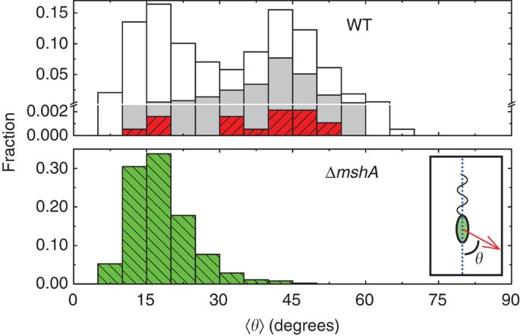Figure 2: Histogram of the trajectory-averaged angular difference (‹θ›) between the direction of motion and the cell-body axis. (Upper) unfilled bars: all mobile WT cells. Grey bars: subset of WT exhibiting orbiting motility. Red bars: subset of WT exhibiting roaming motility. (Lower) ΔmshAmutants. (NWT=1,877,NΔmshA=2,030). (inset) Schematic showing howθis defined. Figure 2: Histogram of the trajectory-averaged angular difference (‹ θ ›) between the direction of motion and the cell-body axis. (Upper) unfilled bars: all mobile WT cells. Grey bars: subset of WT exhibiting orbiting motility. Red bars: subset of WT exhibiting roaming motility. (Lower) Δ mshA mutants. ( N WT =1,877, N Δ mshA =2,030). (inset) Schematic showing how θ is defined. Full size image Hydrodynamic model To elucidate the nature of the interactions between the orbiting and roaming cells and the surface, we turn to theoretical modelling. We consider the hydrodynamic mobilities of both the cell body and the flagellum, solving for the velocities using a force and torque balance. We model the cell body as a half-wavelength of a right-handed helix that rotates CW, while the flagellum rotates counter-CW (CCW) and incorporate interactions between the MSHA pili and the glass surface through a friction coefficient, given by γ (see Methods-Model). The dependence of a trajectory’s radius of curvature ( R curv ) on γ is highly nonlinear. We find that for small γ values, R curv varies quite dramatically with γ , while at larger values of γ the R curv is insensitive to γ . Small values of γ correspond to weak but finite surface interactions. This behaviour of the model describes the roaming phenotype and is consistent with the polydispersity in trajectory curvatures observed for this phenotype. In contrast, larger values of γ produce trajectories with smaller R curv . This behaviour corresponds to the orbiting phenotype, which exhibits relatively monodisperse trajectory curvatures since R curv does not change significantly with increasing γ . A plot of the R curv as a function of γ is shown in Fig. 3a . The model predicts R curv =56 μm when γ =0 and R curv =4 μm when γ =0.1. Example trajectories generated for γ =0.002 and 0.1 are shown in the insets of Fig. 3a , respectively. Due to the distribution of R curv as a function of γ , we expect to see essentially two types of tracks: relatively few low-curvature tracks having polydisperse curvatures and numerous high-curvature tracks having monodisperse curvatures. 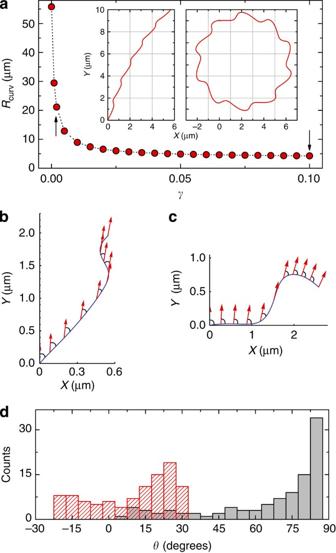Figure 3: Modelled orbital and roaming cell trajectories. (a) Model derived average radius of curvature (Rcurv) as a function of the friction coefficientγ. The arrows indicate two differentγvalues used to model roaming and orbiting phenotypes:γ=0.002 and 0.1, respectively. (inset, left) modelled roaming trajectory for 10 cycles; here,Rcurv=38 μm. (inset, right) Modelled orbiting trajectory for 20 cycles; hereRcurv=7 μm. (b) Magnification of one cycle of the roaming trajectory (froma). (c) Magnification of one cycle of the orbiting trajectory (froma). Arrows indicate the direction of the body axis at discrete points along the track. (d) Histogram of the instantaneousθfor roaming (hatched) and orbiting (filled) over one cycle. Figure 3: Modelled orbital and roaming cell trajectories. ( a ) Model derived average radius of curvature ( R curv ) as a function of the friction coefficient γ . The arrows indicate two different γ values used to model roaming and orbiting phenotypes: γ =0.002 and 0.1, respectively. (inset, left) modelled roaming trajectory for 10 cycles; here, R curv =38 μm. (inset, right) Modelled orbiting trajectory for 20 cycles; here R curv =7 μm. ( b ) Magnification of one cycle of the roaming trajectory (from a ). ( c ) Magnification of one cycle of the orbiting trajectory (from a ). Arrows indicate the direction of the body axis at discrete points along the track. ( d ) Histogram of the instantaneous θ for roaming (hatched) and orbiting (filled) over one cycle. Full size image The phenomenological frictional coefficient γ depends on the interaction strength between the surface and MSHA pili. The strength of this interaction can depend on MSHA pili of specific lengths, heterogeneities on the surface that modulate the interaction strength and the number and distribution of pili on the cell body. Differences between individual cells and chemical and spatial inhomogeneities on the glass surface are expected to result in a range of γ values that can also result in spatial variability. The limiting value of the orbit curvature is fundamental to this problem. In the limit of large γ we find that the minimum radius of curvature is given by where L is the length scale of the cell body and of the flagellum, b is the radius of the flagellum helix, d is the distance from the cell centre to the surface, and 2 r flag and 2 r head are the widths of the flagellum and the cell body, respectively. This simple scaling estimate gives R min ≈4 for the experimentally derived parameters used, which agrees well with the modelled value of 4 μm (see Fig. 3a ) and with the measured value of 3 μm (see Fig. 1g ). Details of the scaling argument are given in the model theory section. Previously reported experimental results for E. coli show that the radius of curvature varies linearly with head size [20] . Although varying the head size could explain some variation in the radius of curvature, the linear relation does not allow for bifurcation into the two distinct motility behaviours we observe in V. cholerae . In petrichously flagellated cells like E. coli , the number of flagella on a cell can influence the width of the helical flagella bundle, which can in turn affect trajectories. However, since V. cholerae has a single polar flagellum, we do not expect a significant influence from these effects. We can calculate the instantaneous value of θ in the model for both trajectories shown in the insets of Fig. 3a . We magnify the first cycle of the trajectory for both motility modes and denote the orientation of the cell body at discrete points with arrows ( Fig. 3b,c ). Here we determine θ at each point as the difference between the arrow and the curve. A histogram of these discrete θ values reveals that orbital cells have a peak around 85° and a mean of 63.6°. Roaming cells have a maximum value near 25° and mean value of 7.4° ( Fig. 3d ). Though the instantaneous θ values for the orbiting cells are high, these values and the trends observed agree with the measured ‹ θ › ( Fig. 2 ). Furthermore, we note that the model generates trajectories with small oscillations combined with a periodic oscillation in speed and θ , in agreement with experiment. The fine structure in the modelled trajectories suggests that the anisotropy of the interactions between the MSHA pili and the surface produces small nutations on the curves due to the rotation of the cell body, which brings MSHA pili into and out of contact with the surface periodically. Although the nutations in the model are more pronounced for orbiting cells, the trajectories for both the orbiting and roaming cells exhibit the predicted nutations ( Fig. 4a ) ( Supplementary Movies 1–3 ). Using heat maps to distinguish instantaneous changes in speed and θ , we observe the periodic changes predicted by our model ( Fig. 4b,c and d,e ). 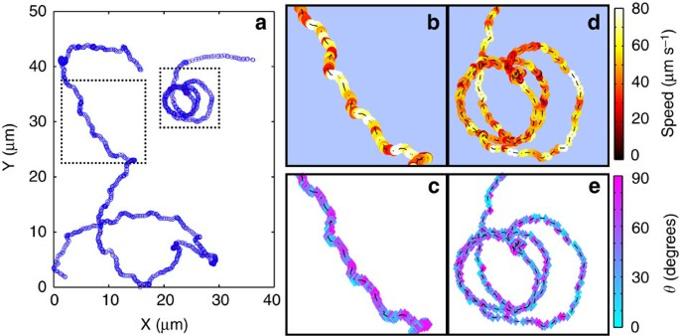Figure 4: Representative roaming and orbiting surface motility trajectories. (a, left) Roaming trajectory. (a, right) Orbiting trajectory. (b) Speed and (c)θheat maps of the boxed region of the roaming trajectory in (a). (d) Speed and (e)θheat maps of the boxed region of the orbital trajectory in (a). Figure 4: Representative roaming and orbiting surface motility trajectories. ( a , left) Roaming trajectory. ( a , right) Orbiting trajectory. ( b ) Speed and ( c ) θ heat maps of the boxed region of the roaming trajectory in ( a ). ( d ) Speed and ( e ) θ heat maps of the boxed region of the orbital trajectory in ( a ). Full size image Pauses and attachment The vast majority of V. cholerae cells that visit the surface within the first few minutes do not attach irreversibly. It is interesting to note that the cells that eventually attach exhibit orbiting motility with a distribution of intermittent pauses during their motion. We define a pause as a displacement smaller than a threshold value of 0.25 μm for a minimum of 25 ms. This threshold distance is greater than 3 × , larger than the uncertainty in determining the centroid of stationary objects, and the duration corresponds to five movie frames. We compare the normalized histograms of pause durations, t pause , for all orbiting and roaming WT cells. During the same period of time orbiting cells exhibit ~30 × more pause events than roaming cells: 9,466 compared with 391. Moreover, roaming cells do not exhibit pauses longer than ~2 s, whereas orbiting cells exhibit a pause distribution with a long ‘statistical tail’ for long pauses, some as long as ~60 s ( Fig. 3a ). We note, however, that the maximum pause times are limited by the length of our high-speed movies and have observed cells that make pauses for ~ O (10) min. To highlight the origin of these pauses, we examine the distribution of pauses for Δ mshA mutants. Both the frequency and duration of pauses in Δ mshA mutants are also significantly lower than that of WT orbiting cells, with almost no pauses longer than ~5 s ( Fig. 5a , middle). We hypothesize that WT surface interactions will change if their MSHA pili could be rendered non binding. Previous studies report the use of methyl α- D -mannopyranoside (dMann), a non-metabolisable sugar that binds to the MSHA pili, to inhibit V. cholerae from adhering and forming biofilms [32] . Importantly, we find that both the frequency and duration of these pauses are strongly suppressed for WT cells incubated in 200 mM dMann. Consistent with this, these cells also exhibit a concomitant attachment defect resulting in a t pause distribution similar to that of Δ mshA ( Fig. 5a , lower). Although unable to attach irreversibly, the dMann incubated WT still exhibit a residual capacity for orbiting and roaming motility, but with shorter surface residence times; this shows that their MSHA pili retain some capability for non-specific interactions to glass [33] . To show this quantitatively, we compare the distribution of surface residence times ( t residence ) of WT cells to dMann incubated WT and to Δ mshA mutants ( Supplementary Fig. S2 ). We find that the t residence distribution for dMann incubated WT represents a middle ground between WT behaviour and Δ mshA behaviour, consistent with finite but attenuated MSHA pili–surface interactions. Taken together, these results suggest that the observed pause distributions arise from MSHA pili–surface interactions and that these events significantly affect irreversible attachment. MSHA pili facilitate adhesion by a hierarchy of effects: In addition to increasing the time spent over surfaces that generate high friction with pili, MSHA pili can directly impact surface attachment by itself. 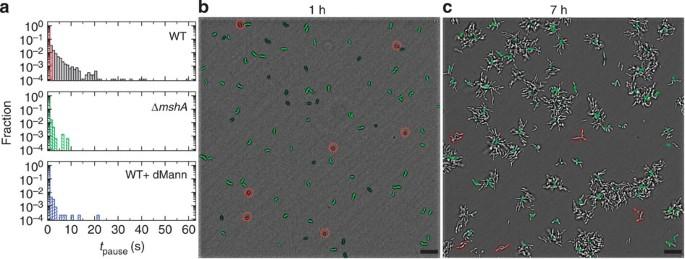Figure 5: Surface-associated pause duration and irreversible attachment. (a) Histogram of pause durations (tpause) for: (Upper) WT orbiting motility mode (grey bars) and roaming motility mode (red hatched bars). (Norbiting=9,466 andNroaming=391); (Middle) ΔmshAmutants (N=1,521); (Lower) WT incubated in 200 mM dMann (NdMann=5,068). (b) False colour image of surface-attached cells 1 h after inoculation. Cells that orbited prior to attachment are shown in light green. Dark green cells attached within the first hour after inoculation, between high-speed movie bursts. The red cells (circled) depart during the subsequent 7 h time-lapse sequence. (c) False colour image of the same field of view 7 h later. We overlay the green cells on the microcolonies to show their origin. Colonies outlined in red were initiated from the bulk during the time lapse. Scale bars, 10 μm. Figure 5: Surface-associated pause duration and irreversible attachment. ( a ) Histogram of pause durations ( t pause ) for: (Upper) WT orbiting motility mode (grey bars) and roaming motility mode (red hatched bars). ( N orbiting =9,466 and N roaming =391); (Middle) Δ mshA mutants ( N =1,521); (Lower) WT incubated in 200 mM dMann ( N dMann =5,068). ( b ) False colour image of surface-attached cells 1 h after inoculation. Cells that orbited prior to attachment are shown in light green. Dark green cells attached within the first hour after inoculation, between high-speed movie bursts. The red cells (circled) depart during the subsequent 7 h time-lapse sequence. ( c ) False colour image of the same field of view 7 h later. We overlay the green cells on the microcolonies to show their origin. Colonies outlined in red were initiated from the bulk during the time lapse. Scale bars, 10 μm. Full size image We combine cell-tracking at the initial stages of V. cholerae surface interaction with time-lapse imaging data to assess the consequences of irreversible attachment enabled by MSHA pili–surface binding ( Fig. 5b,c ). We track attachment across a series of high time-resolution movie bursts taken during the first hour (see Methods) and then monitor microcolony development using time-lapse imaging over many hours (elapsed times~10 h). We computationally colour the attached cells that grow into microcolonies in light and dark green. Cells that orbit prior to attachment are coloured in light green, while cells that attach between high-speed movie bursts are coloured in dark green ( Fig. 5b ). A small number of cells detach and do not participate in the microcolonies that exist at 7 h; these are shown in red. Likewise, a few microcolonies present at the end of the time lapse are seeded by cells that arrive from the bulk fluid during the 7 h window; these are outlined in red ( Fig. 5c ). We note that we do not observe any roaming cells that transition to irreversible attachment directly. By superimposing the sites of initial attachment mediated primarily by orbiting motility onto the locations of eventual microcolonies, we find a large degree of overlap; this can only be true if cells do not exhibit significant surface motility after attachment (see Fig. 5c ). To confirm, we measure the distance from cell-attachment sites to the centre-of-mass of the early microcolonies that these cells form prior to microcolony coalescence. We find that the average separation is 1.1±0.9 μm from three independent time-lapse experiments ( N =249), which is <2 μm average length of a V. cholerae bacterium. In fact, 98% of all surface-attached cells attach within 2.5 μm of the eventual microcolony centre-of-mass (see Supplementary Fig. S3 ). These results indicate that non-swimming surface motility, such as twitching, does not play a major role in V. cholerae microcolony formation. It appears that surface–MSHA pili interactions in V. cholerae largely determine surface attachment sites and ultimately the location of microcolonies. This contrasts sharply with the behaviour of P. aeruginosa : after surface attachment, cells can self-organise into microcolonies that are far from individual cell-attachment sites using exopolysaccharide (EPS)-guided twitching motility [14] . It will be interesting to determine how these differences in surface colonization technologies ultimately relate to bacterial niche diversification. Summary We have shown that MSHA pili–surface interactions strongly affect near-surface swimming of V. cholerae . Our model indicates that surface friction from these interactions generate two distinct motility modes: cells with low friction interactions tend to pass over surfaces by ‘roaming’, whereas cells with high friction interactions tend to loiter above surfaces by ‘orbiting’, and thereby influence the locations of irreversible attachment probabilistically. Our cell-tracking observations suggest that MSHA pili binding to the surface during orbiting motility is a necessary condition for cell motion arrest, and ultimately the transition to irreversible attachment and microcolony formation. Bacteria strains and flow-cell experiment The WT O1 Serotype, El tor Biotype, A1552 strain of V. cholerae and the isogenic mutant strains Δ mshA (lacking MSHA pilin) and Δ flaA (lacking the major flagellin subunit FlaA) were used. The bacteria were cultured in full strength Luria–Bertani (LB) broth overnight under shaking at 30 °C. Prior to inoculation, a subculture was made by diluting the overnight culture into 2% LB (containing 171 mM NaCl), to an optical density at 600 nm (OD 600 ) in the range 0.01–0.03. V. cholerae were then injected into a sterile flow-cell containing the same media and imaged immediately. WT cells used in the dMann experiments were incubated in the same 2% LB containing 200 mM dMann for 45 min prior to inoculation into the flow-cell, which contained the same media. We recorded high-speed movies of V. cholerae motion in the flow-cells with a Phantom V12.1 high-speed camera (Vision Research), collecting ~20,000 bright-field images at 5 ms resolution with a × 100 oil objective on an IX71 Olympus microscope. The series of high-speed movie bursts (see Fig. 5b,c ) were recorded at the same frame rate and duration, and were captured every 4 min during the first 20 min after inoculation. We then recorded a second set of these bursts every 15 min until the end of the first hour. Time-lapse imaging was done using the same flow-cell with an EMCCD camera (Andor iXon) using IQ software (Andor); images were taken once every 10 s for ~10 h. In all experiments, the flow-cell was mounted to a heat-stage on the microscope to maintain a constant temperature of 30 °C. We infused fresh 2% LB starting 1 h after inoculation at a flow rate of 3 ml h −1 . Cell-tracking algorithm and analysis We preprocess every frame of a movie in Matlab (Mathworks) by subtracting the background, scaling, smoothing and thresholding to generate a binary image using Otsu thresholding [34] . Bacteria appear as bright regions. Tracking is done by locating all bright objects that overlap objects in the next frame by combining the two frames into a three-dimensional (3D) matrix and then by locating 3D connected components. We store the results in a tree-like structure with multiple roots [35] ; every newly detected bacterium that appears is recorded as a ‘root’ of the tree. When bacteria interact, they are recorded as a ‘node’ of the tree; when they depart, they are recorded as a ‘leaf’. Each root or node stores the sequence of pixel lists that comprise the bacterium in all frames until the next interaction or detachment event. We measure the instantaneous shape properties of the bacteria using the Matlab regionprops function. From these properties we can calculate the MSD, , where and is the position vector of the j th point on the trajectory and the angled brackets indicate an average over all times t i . The MSD gives information about the average displacement between points in the trajectory separated by a fixed time lag [36] . The instantaneous speed is calculated as, , where Δ t = t i +1 − t i . The angle difference is defined as the angle between a bacterium’s instantaneous velocity and its body axis, limited to the range [13] , [37] . Theoretical modelling We base our model on Lauga et al. [20] , where we consider the hydrodynamic mobilities of the head and the flagellum separately and solve for the velocities using force and torque balance. We assume that the cell does not interact with other cells and is parallel to the no-slip boundary at z =0. We choose the y −axis to lie along the cell axes. The Reynolds number is low, Re ≈10 −4 , so the fluid flow is given by the Stokes equations, which are linear. Therefore, the forces and torques on the cell head and flagellum due to the motion are linear in the velocities and we can write where is the forces and torques acting on part k , and k =head, flag; M k is the mobility matrix of part k ; is the linear and angular velocity of the cell; is the velocity of the rotary motor that rotates the flagellum CCW. V. cholerae have pili on their bodies and as their bodies rotate during swimming, the pili sweep past surfaces. We assume that the pili sweep past the surface once per cycle exerting a time-dependent frictional force on the cell that depends linearly on the instantaneous velocity. The force and torque exerted on the cell due to friction between the pili and the surface is where d is the distance from the surface to the average central position of the head, l is the distance along the cell head from the centre to the longest pili and the phase difference =( l / L −1/2) π , where L is the length of the cell head. We numerically solve for using force and torque balance The pili friction enters the force free condition linearly, however, when we solve for the velocities we invert the sum of mobility matrices and pili friction matrix. After inversion the friction coefficient enters the velocity equations nonlinearly, leading to the nonlinear dependence of the radius of curvature on the friction coefficient. The flagellum is a left-handed helix rotating CCW, described by where 0< s <2 πn . We use resistive force theory (RFT) as an approximation for the mobilities [38] , which were calculated and given in Appendix A of ref. 20 . RFT considers each element δl of filament moving at velocity in a viscous fluid, which is decomposed into the components parallel and perpendicular to the filament, so and each direction is associated with a local drag coefficient c ‖ , c ⊥ . The force on an element of length l is then The resistant coefficients are given by the far field asymptotic results of Katz et al. [39] that consider the effect of a plane boundary: where − b < z ( s )< b is the distance of the helix filament from the helix axis, d is the distance from the surface to the helix axis and r is the radius of the helix filament. The head is approximately half a wavelength of right-handed helix rotating CW, described by where 0< s < π . We use RFT to calculate these mobilities. In our model we use the following values for the parameters, with all distances in micrometres: head length λ h /2=2.2, head rod radius R =0.3, head helix radius B =0.4, gap between surface and the bottom of head h =0.04, height from surface to centre of cell d =0.74, flagellum wavelength λ f =2, number of wavelengths n =3, flagellar helix radius b =0.4, radius of flagellum filament r =0.02 and motor frequency ω =200 Hz. We consider the pili to be concentrated at the leading pole of the cell so l = λ h /4 and =0. We find that the radius of curvature varies with geometric parameters, but we have tried to choose values that are realistic. We also find that the curvature increases with decreasing distance between the cell and the surface, even when keeping the friction coefficient constant. To calculate the radius of curvature, we consider the change in angle Δ θ and x – y displacement Δ ρ of the cell over one rotation of the cell head. By considering the geometry, we have We consider large friction coefficient γ ; in the case where γ →∞ and finite driving torque, the pili must have zero velocity at the point of contact with the surface, so from equation (2) we have where d is the distance from the centre of the cell to the surface. This means that we have rolling motion of the cell head along the surface. Motion in the y -direction is negligible, since U y +Ω x d =0 and Ω x ≪ Ω y . For rolling motion, the displacement of the cell head over one cycle is 2 πd so from equation (8) we have The angular change is Δ θ ~−Ω z Δ t , where Δ t ~1/Δ y , so where, the sign comes from the CW rotation of the cell. In the following we follow the notation of Lauga et al. in ref. 20 , where , is the viscous mobility relating the j th component of velocity or angular velocity, denoted by β , to the i th component of force or torque, denoted by α , for the cell head and flagellum, respectively. Torque balance in the z -direction gives us . From U x =Ω y d and the scaling relations where L and b are the characteristic length and helix radius of both head and flagellum, respectively, we have From an approximate balance of the torques in the y -direction , we have where r head,flag is the width of helix filament of the head and flagellum, and r head >> r flag . Putting this in equation (10) we have We have d > r i , and so the log ratio is O (1). For flagella b/L , d/L ~ O (0.1), so we can use the small angle approximation sin( x )≈ x , so equation (14) becomes With the values we have used in our model and taking a length scale L =4, this scaling argument yields a value R min ≈4, which matches the value R curv =4 that we get in the model for large γ =0.1. The average velocity in the direction towards the surface is 19 μm s −1 when γ =0.1, 12 μm s −1 when γ =0.002 and 2.6 μm s −1 when γ =0. In the model, we assume the distance between the cell and the surface stays constant to leave a gap for the pili, however this velocity difference shows a stronger attraction to the surface in cells with a larger friction coefficient. This is in agreement with the observation that orbiting cells, which correspond to the larger friction coefficients, remain in close proximity to the surface longer than roaming cells or Δ mshA mutants, and that permanently adhered cells originate from the orbiting phenotype. How to cite this article: Utada, A. S. et al. Vibrio cholerae use pili and flagella synergistically to effect motility switching and conditional surface attachment. Nat. Commun. 5:4913 doi: 10.1038/ncomms5913 (2014).